USP11 regulates PML stability to control Notch-induced malignancy in brain tumours The promyelocytic leukaemia (PML) protein controls multiple tumour suppressive functions and is downregulated in diverse types of human cancers through incompletely characterized post-translational mechanisms. Here we identify USP11 as a PML regulator by RNAi screening. USP11 deubiquitinates and stabilizes PML, thereby counteracting the functions of PML ubiquitin ligases RNF4 and the KLHL20–Cul3 (Cullin 3)–Roc1 complex. We find that USP11 is transcriptionally repressed through a Notch/Hey1-dependent mechanism, leading to PML destabilization. In human glioma, Hey1 upregulation correlates with USP11 and PML downregulation and with high-grade malignancy. The Notch/Hey1-induced downregulation of USP11 and PML not only confers multiple malignant characteristics of aggressive glioma, including proliferation, invasiveness and tumour growth in an orthotopic mouse model, but also potentiates self-renewal, tumour-forming capacity and therapeutic resistance of patient-derived glioma-initiating cells. Our study uncovers a PML degradation mechanism through Notch/Hey1-induced repression of the PML deubiquitinase USP11 and suggests an important role for this pathway in brain tumour pathogenesis. The promyelocytic leukaemia (PML) tumour suppressor gene was identified as a target for translocation with retinoic acid receptor-α in acute PML [1] , [2] . The PML protein is an essential component of discrete subnuclear structures called PML nuclear bodies (PML-NBs) [3] , and is a regulator of multiple cellular processes that are altered in cancer, such as proliferation, senescence, cell death and migration [4] , [5] , [6] . PML-knockout mice exhibit enhanced susceptibility to tumorigenesis when challenged with carcinogens [7] or in the context of additional oncogenic events [8] , [9] . In accordance with its tumour suppressive functions, PML protein downregulation is frequently observed in various types of human cancer, including brain tumours [10] . Evidence has emerged that ubiquitin-mediated proteasomal degradation is a key mechanism leading to PML downregulation in tumours [11] . For instance, a CK2-dependent and an E6AP-mediated PML ubiquitination pathway are deregulated in non-small cell lung cancer and Burkitt’s lymphoma, respectively [8] , [12] , [13] , [14] . Recently, we identified a Roc1–Cul3–KLHL20-mediated PML ubiquitination/degradation pathway, which participates in a feedback mechanism to amplify HIF-1 signalling and tumour hypoxia responses. Hyperactivation of this PML degradation pathway is evident in prostate cancer and correlates with disease progression [15] . Despite these findings, it remains undetermined whether PML deubiquitination is abnormally regulated in tumours, as this deubiquitination mechanism has not been identified. In addition to its tumour suppressive functions, PML plays crucial roles in the maintenance and fate determination of stem/progenitor cells. PML loss potentiates proliferation of haematopoietic stem cells (HSCs) [16] and impairs their asymmetric division [17] , leading to HSC exhaustion. PML depletion in mammary progenitor cells increases their proliferation and disturbs the balance of two progenitor populations [18] . During brain neocortical development, PML loss similarly increases the proliferation of neural progenitor cells (NPCs) and compromises their differentiation, thereby skewing the composition of NPC subpopulations [19] . It remains undetermined whether PML exerts similar function in the stem-like cell population of brain tumours and whether PML itself is regulated by core pathways that drive stemness programmes. Glioma is the most common type of primary brain tumour, and glioblastoma multiforme (GBM), a grade IV glioma, is the most common and aggressive glial brain tumour [20] , [21] . The median survival in GBM is 14.6 months with the current standard treatment [22] . Emerging evidence indicates the existence of a subpopulation of tumour cells in glioma with stem cell-like characteristics, referred as glioma-initiating cells (GICs) [23] . GICs exhibit sustained self-renewal and drive tumour initiation, propagation and radio/chemoresistance [24] , [25] , [26] , [27] , [28] . Understanding the mechanisms that govern GIC characteristics is therefore critical to improve therapy for GBM as well as other aggressive cancer types. Notch signalling not only promotes GBM tumour cell proliferation and invasion, but also has a crucial role in maintaining GIC characteristics and supporting GIC niche function [29] , [30] , [31] , [32] , [33] . In this study, we uncover a molecular mechanism linking Notch signalling to PML degradation. We show that Notch acts through Hey1 to repress the expression of USP11, a deubiquitinating (DUB) enzyme for PML. This pathway leads to PML destabilization and is deregulated in GBM. We provide evidence indicating that this pathway promotes multiple malignant features of GBM and GICs. Thus, our study identifies a PML degradation pathway mediated by Notch-induced downregulaton of PML deubiquitinase USP11 and reveals the importance of this pathway in promoting GBM malignancy. USP11 interacts with and stabilizes PML To identify PML-specific DUB, we carried out an unbiased loss-of-function screen using short hairpin RNAs (shRNAs) to individually inhibit the expression of 82 DUBs. HeLa cells transduced with lentivirus carrying these shRNAs were analysed for PML immunofluorescence ( Fig. 1a ). DUBs with two or more shRNAs displaying significant reductions in both PML immunofluorescence and PML-NB number from two independent screens were USP11 and USP40 ( Supplementary Fig. 1a ). They were verified by a secondary screen for the downregulation of PML protein. While USP40 shRNAs did not affect PML expression ( Supplementary Fig. 1b ), knockdown of USP11 by three independent shRNAs induced downregulation of PML protein but not PML messenger RNA ( Fig. 1b ). This downregulation was blocked by proteasome inhibitor MG132 and was accompanied with a decrease of PML protein half-life ( Fig. 1c,d ). Conversely, overexpression of USP11, but not its catalytically dead mutant, elevated PML expression ( Fig. 1e ). USP11 also increased PML half-life ( Fig. 1f ). These data indicate that USP11 upregulates PML by preventing its proteasomal degradation. 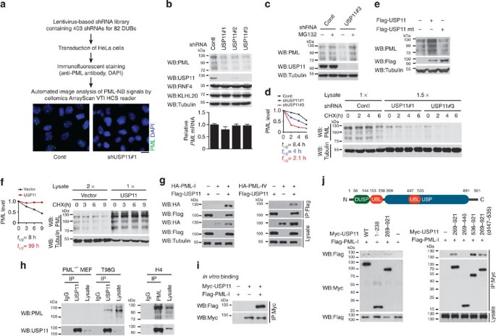Figure 1: USP11 interacts with and stabilizes PML. (a) Schematic presentation of the screening procedure to identify DUBs that regulate PML. Representative images of cells transduced with lentivirus containing control or USP11 shRNA are shown on the bottom. Scale bar, 20 μm. (b) USP11 shRNAs reduce PML protein but not mRNA. HeLa cells transduced with lentivirus carrying USP11 shRNA or control shRNA were analysed by western blot with indicated antibodies (top) or by reverse transcriptase–quantitative PCR (bottom). Data shown are mean±s.d. of three independent experiments. (c) HeLa cells transduced with indicated lentiviruses were treated with 1 μM MG132 for 18 h and analysed by western blot. (d,f) The effects of USP11 knockdown (d) or overexpression (f) on PML half-life. HeLa cells stably expressing indicated shRNAs (d), or U87 cells transfected with indicated constructs (f) were treated with 100 μg ml−1cycloheximide for indicated time periods and were analysed by western blot. The levels of PML relative to that seen at 0 h were quantified and plotted on the left panels and the PML half-life in each cell is indicated on the bottom. (e) Western blot analysis of PML level in HeLa cells transfected with indicated constructs. (g) USP11 interacts with PML-I and PML-IV. Coimmunoprecipitation analysis of 293T cells transfected with indicated constructs. (h) Interaction of endogenous PML with endogenous USP11 in T98G GBM cells and H4 glioma cells was analysed by coimmunoprecipitation. Lysate of PML-null MEFs was used as a control. (i) USP11 and PML interactin vitro. Baculovirally purified USP11 bound on Myc-agarose beads was used to pull down baculovirally purified PML-I. Bound proteins were analysed by western blot with indicated antibodies. (j) Mapping of the USP11 domain involved in PML interaction. The domain organization of USP11 is shown on the top panel. Interaction of PML-I with indicated USP11 mutants in transfected 293T cells was analysed by coimmunoprecipitation (bottom panels). Figure 1: USP11 interacts with and stabilizes PML. ( a ) Schematic presentation of the screening procedure to identify DUBs that regulate PML. Representative images of cells transduced with lentivirus containing control or USP11 shRNA are shown on the bottom. Scale bar, 20 μm. ( b ) USP11 shRNAs reduce PML protein but not mRNA. HeLa cells transduced with lentivirus carrying USP11 shRNA or control shRNA were analysed by western blot with indicated antibodies (top) or by reverse transcriptase–quantitative PCR (bottom). Data shown are mean±s.d. of three independent experiments. ( c ) HeLa cells transduced with indicated lentiviruses were treated with 1 μM MG132 for 18 h and analysed by western blot. ( d , f ) The effects of USP11 knockdown ( d ) or overexpression ( f ) on PML half-life. HeLa cells stably expressing indicated shRNAs ( d ), or U87 cells transfected with indicated constructs ( f ) were treated with 100 μg ml −1 cycloheximide for indicated time periods and were analysed by western blot. The levels of PML relative to that seen at 0 h were quantified and plotted on the left panels and the PML half-life in each cell is indicated on the bottom. ( e ) Western blot analysis of PML level in HeLa cells transfected with indicated constructs. ( g ) USP11 interacts with PML-I and PML-IV. Coimmunoprecipitation analysis of 293T cells transfected with indicated constructs. ( h ) Interaction of endogenous PML with endogenous USP11 in T98G GBM cells and H4 glioma cells was analysed by coimmunoprecipitation. Lysate of PML-null MEFs was used as a control. ( i ) USP11 and PML interact in vitro . Baculovirally purified USP11 bound on Myc-agarose beads was used to pull down baculovirally purified PML-I. Bound proteins were analysed by western blot with indicated antibodies. ( j ) Mapping of the USP11 domain involved in PML interaction. The domain organization of USP11 is shown on the top panel. Interaction of PML-I with indicated USP11 mutants in transfected 293T cells was analysed by coimmunoprecipitation (bottom panels). Full size image As USP11 knockdown did not affect the levels of RNF4 and KLHL20 ( Fig. 1b ), two ubiquitin ligases for PML [15] , [34] , [35] , we determined whether USP11 acts directly on PML. Coimmunoprecipitation analysis revealed that USP11 interacted with both PML-I and PML-IV in transfected cells ( Fig. 1g ). Interaction between endogenous USP11 and endogenous PML was also detected by reciprocal coimmunoprecipitations and the specificity of this interaction was confirmed by using lysates derived from PML -null mouse embryonic fibroblasts (MEFs; Fig. 1h ). Furthermore, purified USP11 and PML-I interacted in vitro ( Fig. 1i ). Domain-mapping analysis revealed that USP11 bound PML through its USP domain ( Fig. 1j ). Within the USP domain, the carboxy-terminal segment encompassing residues 536–921 was responsible for PML interaction. These data support a direct role of USP11 in regulating PML. USP11 deubiquitinates PML We next assessed the effect of USP11 on PML ubiquitination. USP11 knockdown increased the amount of PML-I modified by haemagglutinin (HA)-ubiquitin ( Fig. 2a ). A similar result was obtained with another PML isoform, PML-IV ( Fig. 2b ). Purification of ubiquitinated proteins under denaturing conditions followed by western blot analysis of PML further demonstrated the elevation of polyubiquitin modification on endogenous PML in USP11-knockdown cells ( Fig. 2c ). In the reciprocal experiment, overexpression of USP11, but not its catalytically inactive mutant, reduced PML ubiquitination ( Fig. 2d ). Next, we determined whether USP11 could deubiquitinate PML in vitro . To this end, recombinant PML-I was first subjected to an in vitro ubiquitination assay in the presence of E1, E2 and baculovirally purified Roc1–Cul3–KLHL20 E3 ligase complex, and the resulting product was incubated with baculovirally purified USP11 or its catalytically dead mutant. We found that the polyubiquitin chain on PML generated by in vitro ubiquitination was efficiently removed by USP11, but not its mutant ( Fig. 2e ). These findings collectively support that PML is a direct and physiological substrate of USP11. 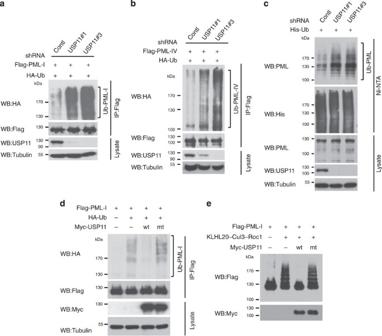Figure 2: USP11 deubiquitinates PML and antagonizes the function of PML ubiquitin ligases. (a,b) USP11 shRNAs increase the ubiquitination levels of PML-I (a) and PML-IV (b). Immunoprecipitation and/or western blot analysis of 293T cells transduced with lentivirus expressing control or USP11 shRNAs and transfected with indicated constructs. (c) Tandem affinity purification of ubiquitinated endogenous PML under denaturing conditions form U87 cells transduced with lentivirus expressing control or USP11 shRNAs and transfected with His-ubiquitin. (d) USP11 decreases PML-I ubiquitinationin vivo. PML-I ubiquitination in 293T cells transfected with indicated constructs was analysed as ina. (e)In vitrodeubiquitination of PML by USP11. Purified PML-I was subjected toin vitroubiquitination reaction in the presence of E1, E2 and Roc1–Cul3–KLHL20 complex and the resulting products were incubated with baculovirally purified USP11 or its mutant for deubiquitination (Methods). The reaction products were examined by western blot with indicated antibodies. Figure 2: USP11 deubiquitinates PML and antagonizes the function of PML ubiquitin ligases. ( a , b ) USP11 shRNAs increase the ubiquitination levels of PML-I ( a ) and PML-IV ( b ). Immunoprecipitation and/or western blot analysis of 293T cells transduced with lentivirus expressing control or USP11 shRNAs and transfected with indicated constructs. ( c ) Tandem affinity purification of ubiquitinated endogenous PML under denaturing conditions form U87 cells transduced with lentivirus expressing control or USP11 shRNAs and transfected with His-ubiquitin. ( d ) USP11 decreases PML-I ubiquitination in vivo . PML-I ubiquitination in 293T cells transfected with indicated constructs was analysed as in a . ( e ) In vitro deubiquitination of PML by USP11. Purified PML-I was subjected to in vitro ubiquitination reaction in the presence of E1, E2 and Roc1–Cul3–KLHL20 complex and the resulting products were incubated with baculovirally purified USP11 or its mutant for deubiquitination (Methods). The reaction products were examined by western blot with indicated antibodies. Full size image USP11 opposes the effects of PML ubiquitin ligases PML ubiquitination can be catalysed by RNF4 or the Roc1–Cul3–KLHL20 complex. While the former specifically targets sumoylated PML [34] , [35] , the latter does not distinguish sumoylated from unmodified PML [15] . Remarkably, USP11 was able to antagonize RNF4- and Roc1–Cul3–KLHL20-mediated PML ubiquitination in 293T cells and GBM cell line U87 ( Supplementary Fig. 2a,b ). Consistent with a role in counteracting the function of RNF4, USP11 prevented the degradation of sumoylated PML in As 2 O 3 -treated cells ( Supplementary Fig. 2c ). However, since USP11 was also capable of targeting PML ubiquitinated by KLHL20-containing E3 ligase, its function was not restricted to sumoylated PML and could efficiently deubiquitinate a sumoylation-defective mutant of PML, PML-I-3KR [34] ( Supplementary Fig. 2d ). Furthermore, under normal growth conditions, USP11 upregulated both sumoylated and unmodified PML ( Supplementary Fig. 2e ). Our results collectively indicate that USP11 possesses a broad specificity to catalyse PML modified by RNF4 or the Roc1–Cul3–KLHL20 complex. USP11-mediated PML stabilization blocks GBM malignant traits Next, we investigated whether USP11-mediated PML deubiquitination is impaired in certain tumours to result in PML degradation. Analysis of the Genevestigator database revealed that USP11 mRNA was abundantly expressed in the brain of normal human tissues ( Supplementary Fig. 3a ). By searching the Repository for Molecular Brain Neoplasia Data (REMBRANDT) database, which contains microarray-derived gene expression data from patients with malignant glioma, we found that USP11 mRNA was downregulated in glioma relative to non-tumour brain tissues, with the grade IV GBM showing the highest extent of downregulation ( Supplementary Fig. 3b ). We therefore assessed the influence of USP11-dependent PML stabilization on the hallmarks of GBM. For this purpose, we infected GBM cell line U251 with lentivirus carrying USP11. This overexpression of USP11 increased PML levels ( Fig. 3a ) and decreased several GBM malignant traits, such as cell proliferation, migration and invasion ( Fig. 3b ). To demonstrate that these tumour-suppressing functions of USP11 resulted from PML upregulation, the USP11-overexpressing cells were infected with lentivirus carrying PML shRNA to reduce PML expression to a level comparable to that in control cells ( Fig. 3a ). Remarkably, this PML knockdown completely abrogated these tumour-suppressing effects of USP11 ( Fig. 3b ). In the reciprocal experiment, USP11 depletion in a low-grade glioma cell line H4 not only reduced PML levels but also promoted cell proliferation, migration and invasion ( Fig. 3c,d ). Knockdown of PML phenocopied the effects of USP11 knockdown. Furthermore, these tumour-promoting effects of USP11 shRNAs were completely blocked by expression of an shRNA-resistant USP11, thus demonstrating the specificity of USP11 shRNA. More importantly, the effects of USP11 shRNAs were also reversed by overexpression of PML-IV. Of note, PML-IV was used in this experiment as it elicited stronger tumour suppressive effects than PML-I ( Supplementary Fig. 3c ). Altogether, these data indicate that USP11-dependent PML stabilization suppresses multiple malignant traits of GBM. 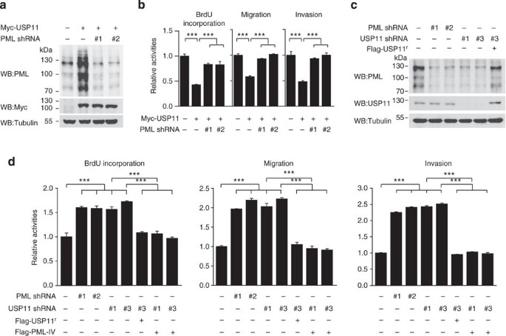Figure 3: USP11-mediated PML stabilization inhibits glioma cell migration and invasion. (a) Western blot analysis of USP11 and PML expression in U251 cells transduced with lentivirus carrying control (−) or PML shRNA and/or USP11 expression construct. (b) Proliferation, migration and invasion capabilities of U251 cells as ina. (c) Western blot analysis of USP11 and PML expression in H4 cells transduced with lentivirus carrying control (−) or indicated shRNAs and/or resistant USP11 (USP11r) construct. (d) H4 cells as incwere transduced with or without lentivirus carrying PML-IV and assayed for proliferation, migration and invasion. Data in panelsbanddare mean±s.d. (***P<0.001 byt-test) of three independent experiments. Figure 3: USP11-mediated PML stabilization inhibits glioma cell migration and invasion. ( a ) Western blot analysis of USP11 and PML expression in U251 cells transduced with lentivirus carrying control (−) or PML shRNA and/or USP11 expression construct. ( b ) Proliferation, migration and invasion capabilities of U251 cells as in a . ( c ) Western blot analysis of USP11 and PML expression in H4 cells transduced with lentivirus carrying control (−) or indicated shRNAs and/or resistant USP11 (USP11 r ) construct. ( d ) H4 cells as in c were transduced with or without lentivirus carrying PML-IV and assayed for proliferation, migration and invasion. Data in panels b and d are mean±s.d. (*** P <0.001 by t -test) of three independent experiments. Full size image Hey1 upregulation and USP11/PML downregulation in GBM Having demonstrated a tumour suppressive role of USP11 in GBM, we next determined the aetiology of USP11 mRNA downregulation in this type of cancer. To address whether USP11 is transcriptionally repressed in GBM, we utilized the PROMO 3.0 program to predict transcription factor-binding sites and searched chromatin immunoprecipitation (ChIP)-seq databases via the UCSC Genome Browser to uncover transcription factors bound on the USP11 promoter. Among these candidates, we focused on factors with transcriptional repression capabilities. We then searched the REMBRANDT database to evaluate whether these transcriptional repressors are upregulated in GBM and whether their upregulation correlates with USP11 downregulation. Among transcription factors that satisfied these criteria, we were particularly interested in Hey1 because it elicits an opposite effect relative to PML on NPC maintenance [19] , [36] . Furthermore, previous studies demonstrated that Hey1 is upregulated in glioma and its overexpression correlates with high-grade glioma and poor patient survival [37] , [38] . To validate the clinical relevance of Hey1 in GBM and the correlation of its expression with USP11 and PML expression, we performed immunohistochemistry (IHC) analysis on tissues derived from a cohort of glioma patients. Representative IHC data from a grade II specimen and a grade IV specimen were presented in Fig. 4a . By analysing specimens from all patients, we found that grade IV GBM exhibited significant higher expression of Hey1 and lower expression of USP11 and PML, in comparison with the grade II/III patients ( Fig. 4b ). Furthermore, Hey1 expression correlated inversely with USP11 and PML expression, whereas USP11 expression correlated positively with PML expression ( Fig. 4c ). These data strongly suggest the existence of a Hey1/USP11/PML pathway in glioma and the association of its hyperactivation with GBM. 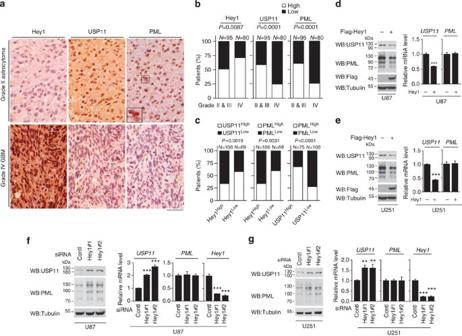Figure 4: Hey1 downregulates USP11 and PML in GBM. (a) Representative IHC staining for Hey1, USP11 and PML in consecutive slides derived from a grade II astrocytoma specimen and a grade IV GBM specimen. Scale bar, 50 μm. The boxed area is enlarged to show in the inset for visualizing PML-NBs. (b) Summary of the Hey1, USP11 and PML expression profiles in 95 grade II/III and 80 grade IV glioma patients. (c) Correlations among the Hey1, USP11 and PML expression levels in the cohort of 175 glioma patients. ThePvalues in panelsbandcwere calculated by Fisher’s exact test. (d) Western blot (left panels) and reverse transcriptase (RT)–quantitative PCR (qPCR; right panels) analysis of USP11 and PML expression in U87 cells transfected with Hey1. (e) Western blot and RT–qPCR analysis of USP11 and PML expression in U251 cells transfected with Hey1. (f) Western blot and RT–qPCR analysis in U87 cells transfected with Hey1 siRNAs. (g) Western blot and RT–qPCR analysis in U251 cells transfected with Hey1 siRNAs. Data in panelsd–gare mean±s.d. (**P<0.01 and ***P<0.001 byt-test) of three independent experiments. Figure 4: Hey1 downregulates USP11 and PML in GBM. ( a ) Representative IHC staining for Hey1, USP11 and PML in consecutive slides derived from a grade II astrocytoma specimen and a grade IV GBM specimen. Scale bar, 50 μm. The boxed area is enlarged to show in the inset for visualizing PML-NBs. ( b ) Summary of the Hey1, USP11 and PML expression profiles in 95 grade II/III and 80 grade IV glioma patients. ( c ) Correlations among the Hey1, USP11 and PML expression levels in the cohort of 175 glioma patients. The P values in panels b and c were calculated by Fisher’s exact test. ( d ) Western blot (left panels) and reverse transcriptase (RT)–quantitative PCR (qPCR; right panels) analysis of USP11 and PML expression in U87 cells transfected with Hey1. ( e ) Western blot and RT–qPCR analysis of USP11 and PML expression in U251 cells transfected with Hey1. ( f ) Western blot and RT–qPCR analysis in U87 cells transfected with Hey1 siRNAs. ( g ) Western blot and RT–qPCR analysis in U251 cells transfected with Hey1 siRNAs. Data in panels d – g are mean±s.d. (** P <0.01 and *** P <0.001 by t -test) of three independent experiments. Full size image Hey1 represses USP11 to downregulate PML Next, we investigated whether Hey1 could regulate the expression of USP11 and PML. Overexpression of Hey1 in GBM cell lines U87 decreased USP11 mRNA and protein ( Fig. 4d ). Consistent with the regulation of PML protein stability by USP11, Hey1-induced USP11 downregulation resulted in a concomitant reduction of PML protein but not mRNA. Similar results were obtained with another GBM cell line, U251 ( Fig. 4e ). In the reciprocal experiments, Hey1 knockdown in U87 and U251 cells upregulated USP11 mRNA, USP11 protein and PML protein, but not PML mRNA ( Fig. 4f,g ). Hey1 overexpression and knockdown also decreased and increased the number of PML-NBs, respectively ( Supplementary Fig. 4a,b ). These findings demonstrated a role of Hey1 in downregulation of USP11 and PML. Hey1 acts as a corepressor on the USP11 promoter To explore the mechanism of Hey1-induced USP11 downregulation, we analysed the 5′-regulatory region of USP11 ( Fig. 5a ). Using a set of ChIP primers, we found that Flag-Hey1 bound to a region 3′ to the transcriptional start site of USP11 gene ( Fig. 5b ), which is consistent with data retrieved from the ChIP-seq database. Endogenous Hey1 also bound to this region and the binding was not detected in Hey1-knockdown cells ( Fig. 5c ), thus demonstrating the specificity of ChIP analysis. Using luciferase reporter assay, we found that Hey1 repressed the USP11 promoter activity and that the +171/+335 (0.16K) region of USP11 promoter was responsible for this repression ( Fig. 5d ). Although this region contains two E boxes, the preferred binding sites for Hey1, their disruption did not affect Hey1-induced repression. Since an Sp1-like factor was reported to cooperate with Hey1 in transcription [39] , we investigated the role of several Sp1-binding sites found in this region. Importantly, Hey1-induced repression of USP11 was abrogated partially by mutating either of the first two Sp1 sites and completely by disrupting both ( Fig. 5d ), suggesting that Hey1 acts through Sp1-binding sites to repress USP11. Consistent with this notion, endogenous Sp1 was recruited to the Hey1-binding region of USP11 promoter ( Fig. 5e ) and Sp1 depletion abolished Hey1 recruitment to this region ( Fig. 5f ). Furthermore, re-ChIP analysis demonstrated the formation of Sp1–Hey1 complex on the USP11 promoter ( Fig. 5g ). All of these findings support a corepressor function of Hey1 in regulating USP11 promoter activity. In contrast to this function of Hey1, Sp1 depletion did not significantly alter USP11 promoter activity, although it abrogated the effect of Hey1 short interfering RNA (siRNA; Fig. 5h ). These findings suggest a dual role of Sp1 in regulating USP11 transcription and Hey1 binding switches the function of Sp1 from an activator to a repressor ( Fig. 5i ). 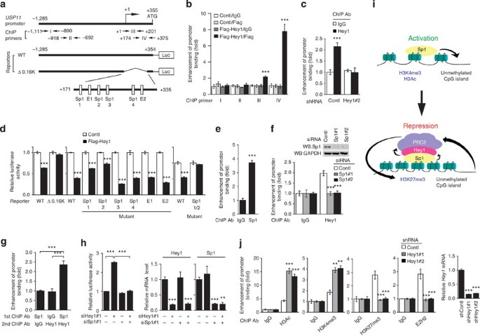Figure 5: Sp1 recruits Hey1 to theUSP11promoter to induce transcriptional repression. (a) Schematic representation of the 5′-regulatory region ofUSP11gene, the luciferase reporter and the ChIP primers used in this study. The positions of two E boxes and four Sp1-binding regions are indicated. (b) qChIP assay in U87 cells transfected with control vector or Flag-Hey1 using control IgG or anti-Flag antibody for immunoprecipitation and indicated primer set for quantitative PCR. (c) qChIP analysis in U87 cells stably expressing indicated shRNAs using control IgG or Hey1 antibody for immunoprecipitation. Primer set IV was used for qChIP assays thereafter. (d) Reporter activity assay of U87 cells transfected with control vector or Flag-Hey1 together with indicated reporter constructs. The luciferase activities in the Flag-Hey1-expressing cells were normalized with those in the control cells. (e) qChIP analysis in U87 cells with control or Sp1 antibody. (f) qChIP analysis in U87 cells expressing control or Sp1 shRNAs with indicated antibodies. The expression levels of Sp1 protein are shown on the top. (g) Re-ChIP analysis in U87 cells with indicated antibodies. (h) Promoter activity assay of U87 cells transfected with the wild-type luciferease reporter construct shown inatogether with indicated siRNAs. The relativeHey1andSp1mRNA levels in each group are shown on the right. (i) A model for the mechanism by which Hey1 repressesUSP11transcription (see text). (j) qChIP analysis in U87 cells transfected with Hey1 shRNAs with indicated antibodies. Data in all panels are mean±s.d. (**P<0.01 and ***P<0.001 byt-test) of three independent experiments. Figure 5: Sp1 recruits Hey1 to the USP11 promoter to induce transcriptional repression. ( a ) Schematic representation of the 5′-regulatory region of USP11 gene, the luciferase reporter and the ChIP primers used in this study. The positions of two E boxes and four Sp1-binding regions are indicated. ( b ) qChIP assay in U87 cells transfected with control vector or Flag-Hey1 using control IgG or anti-Flag antibody for immunoprecipitation and indicated primer set for quantitative PCR. ( c ) qChIP analysis in U87 cells stably expressing indicated shRNAs using control IgG or Hey1 antibody for immunoprecipitation. Primer set IV was used for qChIP assays thereafter. ( d ) Reporter activity assay of U87 cells transfected with control vector or Flag-Hey1 together with indicated reporter constructs. The luciferase activities in the Flag-Hey1-expressing cells were normalized with those in the control cells. ( e ) qChIP analysis in U87 cells with control or Sp1 antibody. ( f ) qChIP analysis in U87 cells expressing control or Sp1 shRNAs with indicated antibodies. The expression levels of Sp1 protein are shown on the top. ( g ) Re-ChIP analysis in U87 cells with indicated antibodies. ( h ) Promoter activity assay of U87 cells transfected with the wild-type luciferease reporter construct shown in a together with indicated siRNAs. The relative Hey1 and Sp1 mRNA levels in each group are shown on the right. ( i ) A model for the mechanism by which Hey1 represses USP11 transcription (see text). ( j ) qChIP analysis in U87 cells transfected with Hey1 shRNAs with indicated antibodies. Data in all panels are mean±s.d. (** P <0.01 and *** P <0.001 by t- test) of three independent experiments. Full size image We next investigated whether Hey1 recruitment alters chromatin structure to result in transcriptional repression. Remarkably, Hey1 depletion increased USP11 promoter-associated H3 acetylation and H3K4 trimethylation and reduced H3K27 trimethylation and recruitment of EZH2, the histone methyltransferase for H3K27 trimethylation ( Fig. 5j ). Altogether, our data indicate that Sp1 is responsible for the recruitment of corepressor Hey1 to the USP11 promoter. Hey1 occupancy leads to chromatin compaction and transcriptional repression through a further recruitment of the histone modifier PRC2 complex ( Fig. 5i ). Notch induces Hey1 to downregulate USP11 and PML Hey1 is a downstream effector of Notch [40] , [41] . Accordingly, overexpression of constitutively active Notch (Notch intracellular domain, referred as NIC) in U87 and U251 cells downregulated USP11 and PML expression ( Fig. 6a,b ). Conversely, inactivation of Notch by treatment of U87 and U251 cells with a γ-secretase inhibitor N-[N-(3,5-difluorophenacetyl)-L-alanyl]-S-phenylglycine t-butyl ester (DAPT) increased USP11 and PML expression. Furthermore, depletion of Notch1 by two independent siRNAs also increased USP11 and PML expression ( Fig. 6c ). We also observed that NIC or Hey1 overexpression in U87 and U251 cells elevated PML ubiquitination ( Fig. 6d ), whereas DAPT inhibited PML ubiquitination ( Fig. 6e ). Importantly, the NIC-induced PML ubiquitination was abrogated by Hey1 depletion or USP11 overexpression ( Fig. 6f ). Finally, the NIC-induced PML downregulation was reversed by proteasome inhibitor MG132 ( Fig. 6g ). These results establish a link between USP11 and Notch and uncover a Notch/Hey1-induced PML degradation pathway in GBM. 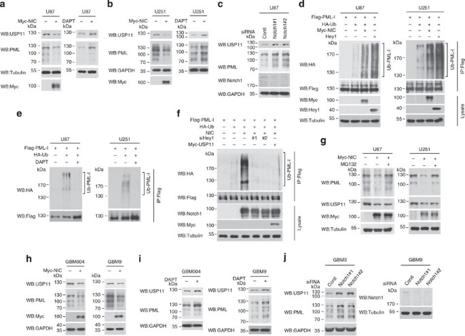Figure 6: Notch acts upstream of Hey1 to induce USP11 and PML downregulation. (a) Western blot analysis of USP11 and PML expression in U87 cells transfected with NIC (left) or treated with 10 μM DAPT for 36 h (right). (b) Western blot analysis of USP11 and PML expression in U251 cells transfected with NIC (left) or treated with 10 μM DAPT for 36 h (right). (c) Western blot analysis of USP11, PML and Notch1 expression in U87 cells transfected with indicated siRNAs. (d) Immunoprecipitation and western blot analysis of PML-I ubiquitination in U87 and U251 cells transfected with indicated constructs. (e) Immunoprecipitation and western blot analysis of PML-I ubiquitination in U87 and U251 cells transfected with indicated constructs and treated with or without DAPT. (f) Immunoprecipitation and western blot analysis of PML-I ubiquitination in U87 and U251 cells transfected with indicated constructs and siRNA. (g) Western blot analysis of USP11 and PML expression in U87 or U251 cells transfected with NIC and treated with 1 μM MG132 for 18 h. (h) Western blot analysis of USP11 and PML expression in indicated GICs transfected with NIC. (i) Western blot analysis of USP11 and PML expression in indicated GICs treated with DAPT. (j) Western blot analysis of USP11, PML and Notch1 expression in indicated GICs transfected with Notch1 siRNAs. Figure 6: Notch acts upstream of Hey1 to induce USP11 and PML downregulation. ( a ) Western blot analysis of USP11 and PML expression in U87 cells transfected with NIC (left) or treated with 10 μM DAPT for 36 h (right). ( b ) Western blot analysis of USP11 and PML expression in U251 cells transfected with NIC (left) or treated with 10 μM DAPT for 36 h (right). ( c ) Western blot analysis of USP11, PML and Notch1 expression in U87 cells transfected with indicated siRNAs. ( d ) Immunoprecipitation and western blot analysis of PML-I ubiquitination in U87 and U251 cells transfected with indicated constructs. ( e ) Immunoprecipitation and western blot analysis of PML-I ubiquitination in U87 and U251 cells transfected with indicated constructs and treated with or without DAPT. ( f ) Immunoprecipitation and western blot analysis of PML-I ubiquitination in U87 and U251 cells transfected with indicated constructs and siRNA. ( g ) Western blot analysis of USP11 and PML expression in U87 or U251 cells transfected with NIC and treated with 1 μM MG132 for 18 h. ( h ) Western blot analysis of USP11 and PML expression in indicated GICs transfected with NIC. ( i ) Western blot analysis of USP11 and PML expression in indicated GICs treated with DAPT. ( j ) Western blot analysis of USP11, PML and Notch1 expression in indicated GICs transfected with Notch1 siRNAs. Full size image To determine whether the Notch/Hey1-dependent PML degradation pathway exists in GICs, we utilized two primary GBM patient-derived initiating cells, GBM9 and GBM004. Overexpression of NIC in each GIC reduced USP11 and PML ( Fig. 6h ), whereas γ-secretase inhibitor or Notch1 siRNA increased USP11 and PML ( Fig. 6i,j ). Thus, the Notch/Hey1/USP11/PML pathway is manifested in GICs. Notch/Hey1/USP11/PML axis promotes aggressive GBM behaviours Next, we evaluated the impact of Notch-induced PML degradation pathway on GBM malignancy. For this purpose, we established a set of stable cell lines derived from U251 ( Fig. 7a ). Consistent with the proliferation effect of Notch on GBM, DAPT significantly reduced the proliferation of parental U251 cells ( Fig. 7b ). Importantly, this effect was completely blocked by Hey1 overexpression, USP11 depletion or PML depletion. Similar findings were observed with another GBM cell line, U87 ( Supplementary Fig. 5a,b ). Conversely, activation of this PML degradation pathway by Hey1 overexpression, USP11 depletion or PML depletion in U87 and U251 cells enhanced the proliferation and soft agar colony formation activities and the effects of Hey1 overexpression or USP11 depletion were blocked by PML-IV overexpression ( Fig. 7c,d and Supplementary Fig. 5c,d ). These data support a role of Notch/Hey1-induced PML degradation pathway in GBM proliferation and transformation. 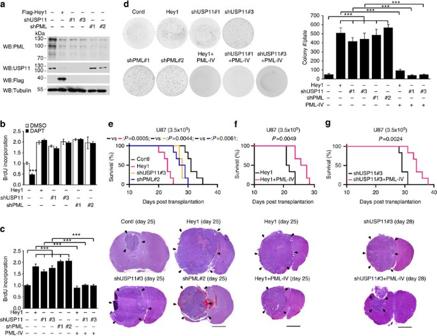Figure 7: Notch/Hey1-induced PML degradation pathway promotes GBM malignant phenotypes. (a) Western blot analysis of PML and USP11 expression levels in U251 derivatives. These stable lines were used in experiments shown in panelsb–d. (b) Proliferation assay of U251 derivatives treated with or without 10 μM DAPT. (c) Proliferation assay of U251 derivatives as indicated. (d) Soft agar colony formation assay of U251 derivatives. Representative images are shown on the left and quantitative data are on the right. Data in panelsb–dare mean±s.d. (***P<0.001 byt-test of three independent experiments). (e–g) Kaplan–Meier survival curves of mice implanted with U87 cells stably expressing indicated constructs (upper panels),n=6 mice for each indicated cell line. ThePvalues were determined by log-rank test. Representative light micrographs of brain tumours formed at indicated days after implantation are shown on the bottom panels. Brain tumours are marked by arrows. Scale bars, 2 mm. The expression levels of USP11 and PML in the U87 derivatives are shown inSupplementary Fig. 5a. Figure 7: Notch/Hey1-induced PML degradation pathway promotes GBM malignant phenotypes. ( a ) Western blot analysis of PML and USP11 expression levels in U251 derivatives. These stable lines were used in experiments shown in panels b – d . ( b ) Proliferation assay of U251 derivatives treated with or without 10 μM DAPT. ( c ) Proliferation assay of U251 derivatives as indicated. ( d ) Soft agar colony formation assay of U251 derivatives. Representative images are shown on the left and quantitative data are on the right. Data in panels b – d are mean±s.d. (*** P <0.001 by t -test of three independent experiments). ( e – g ) Kaplan–Meier survival curves of mice implanted with U87 cells stably expressing indicated constructs (upper panels), n =6 mice for each indicated cell line. The P values were determined by log-rank test. Representative light micrographs of brain tumours formed at indicated days after implantation are shown on the bottom panels. Brain tumours are marked by arrows. Scale bars, 2 mm. The expression levels of USP11 and PML in the U87 derivatives are shown in Supplementary Fig. 5a . Full size image To demonstrate the role of Notch/Hey1-induced PML degradation in brain tumour growth in vivo , we intracranially injected U87 derivatives into nude mice. Mice injected with cells expressing Hey1, USP11 shRNA or PML shRNA exhibited larger brain tumours and shorter survival compared with those injected with control cells ( Fig. 7e ). Furthermore, PML-IV overexpression suppressed both Hey1-driven and USP11 shRNA-driven tumour growth and prolonged survival ( Fig. 7f,g ). Our findings uncover a key role of Notch/Hey1-induced PML degradation pathway in brain tumour growth in vivo . Notch/Hey1/USP11/PML axis potentiates GIC characteristics We next investigated the impacts of the Notch/Hey1-induced PML degradation pathway on the biology of GICs. First, we tested the self-renewal capability of GICs by sphere formation assay. As expected, DAPT treatment of GBM9 cells reduced neurosphere number and size. Importantly, Hey1 overexpression, USP11 depletion or PML depletion each rescued this effect of DAPT ( Fig. 8a ). Similar results were observed with another GIC, GBM004 ( Supplementary Fig. 6a ). We further showed that NIC or Hey1 overexpression in GBM9 and GBM004 cells potentiated self-renewal activity and these effects were abolished by USP11 or PML-I overexpression ( Fig. 8b and Supplementary Fig. 6b ). Of note, PML-I was used in this case because it elicited a stronger effect than PML-IV on suppressing neurosphere formation ( Supplementary Fig. 6c ). In the reciprocal experiment, depletion of Hey1 in GBM9 and GBM004 cells diminished the number and size of neurospheres, which were reversed by PML depletion ( Fig. 8c and Supplementary Fig. 6d ). These data provide substantial evidence for the role of Notch/Hey1-induced PML degradation pathway in promoting the self-renewal capability of GICs. 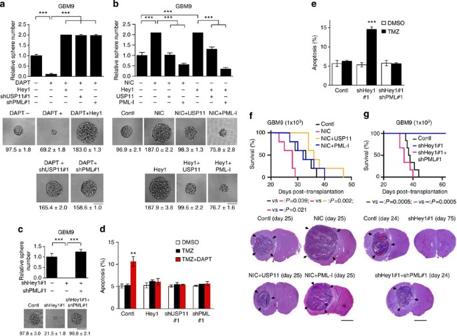Figure 8: Notch/Heyl-induced PML degradation pathway promotes GIC characteristic. (a) Neurosphere-forming abilities of GBM9 cells stably expressing indicated constructs. (b) Neurosphere-forming abilities of GBM9 cells stably expressing indicated constructs. (c) Neurosphere-forming abilities of GBM9 cells stably expressing indicated constructs. For panels (a–c), representative images of GIC neurospheres and their diameters (represented as mean±s.d. of three independent experiments, 30 neurospheres per group per experiment) are indicated on the bottom. Scale bars, 100 μm. (d) Effect of Notch-induced PML degradation pathway on the chemoresistant character of GICs. Apoptosis assay of GBM9 cells stably expressing indicated constructs and treated with TMZ and/or DAPT as described in Methods. (f) Apoptosis assay of GBM9 cells stably expressing indicated constructs and treated with TMZ. (f,g) Kaplan–Meier survival curves (upper panels) of mice implanted with 1 × 103GBM9 cells stably expressing indicated constructs,n=5 mice (f) andn=6 mice (g) for each indicated cell line (upper panels). ThePvalues were determined by log-rank test. Representative light micrograph of brain tumours formed at indicated days after implantation are shown on the bottom panels. Brain tumours are marked by arrows. Scale bars, 2 mm. Data in panelsa–eare mean±s.d. (**P<0.01 byt-test,***P<0.001) of three independent experiments. Figure 8: Notch/Heyl-induced PML degradation pathway promotes GIC characteristic. ( a ) Neurosphere-forming abilities of GBM9 cells stably expressing indicated constructs. ( b ) Neurosphere-forming abilities of GBM9 cells stably expressing indicated constructs. ( c ) Neurosphere-forming abilities of GBM9 cells stably expressing indicated constructs. For panels ( a – c ), representative images of GIC neurospheres and their diameters (represented as mean±s.d. of three independent experiments, 30 neurospheres per group per experiment) are indicated on the bottom. Scale bars, 100 μm. ( d ) Effect of Notch-induced PML degradation pathway on the chemoresistant character of GICs. Apoptosis assay of GBM9 cells stably expressing indicated constructs and treated with TMZ and/or DAPT as described in Methods. ( f ) Apoptosis assay of GBM9 cells stably expressing indicated constructs and treated with TMZ. ( f , g ) Kaplan–Meier survival curves (upper panels) of mice implanted with 1 × 10 3 GBM9 cells stably expressing indicated constructs, n =5 mice ( f ) and n =6 mice ( g ) for each indicated cell line (upper panels). The P values were determined by log-rank test. Representative light micrograph of brain tumours formed at indicated days after implantation are shown on the bottom panels. Brain tumours are marked by arrows. Scale bars, 2 mm. Data in panels a – e are mean±s.d. (** P <0.01 by t -test,*** P <0.001) of three independent experiments. Full size image Notch signaling is known to confer chemoresistance of GICs [42] . Accordingly, DAPT sensitized GBM9 cells to temozolomide (TMZ), a standard cytotoxic agent for treating GBM [22] . The chemosensitizing effect of DAPT was abrogated by Hey1 overexpression, USP11 depletion or PML depletion ( Fig. 8d ). In the reciprocal experiment, Hey1 silencing sensitized GBM9 cells to TMZ, which was reversed by PML depletion ( Fig. 8e ). These findings support the idea that Hey1-induced USP11 and PML downregulation mediates the chemoresistant effect of Notch. Next, we determined the role of Notch-induced PML degradation in the tumour-forming ability of GICs by intracranially injecting a small number of tumour cells to the nude mice. Mice injected with the NIC-expressing GBM9 cells formed larger brain tumours and survived shorter than mice injected with GBM9 cells carrying control vector. This effect of NIC was suppressed by co-expression of USP11 or PML-I ( Fig. 8f ). Conversely, Hey1 shRNA significantly suppressed the tumour-forming ability of GBM9 cells and this effect was reversed by PML depletion ( Fig. 8g ). Our data strongly support a role for the Notch-induced PML degradation pathway in promoting the tumour-forming ability of GICs. PML is a major effector of Notch/Hey1/USP11 axis in GBM To corroborate that the effects of Notch/Hey1/USP11 axis on GBM and GICs are dependent on PML ubiquitination/degradation, we sought to generate a USP11-resistant mutant of PML. By analysing a panel of PML deletion mutants, we found that residues 327–344 of PML was the minimal region required for USP11 interaction ( Fig. 9a,b ). In line with this finding, ubiquitination of the PMLd327-344 mutant was no longer regulated by USP11, NIC or Hey1, which was in sharp contrast to the wild-type PML ( Fig. 9c,d ). Consequently, NIC- or Hey1-induced downregulation and USP11-induced upregulation of PML were completely abolished by this deletion ( Fig. 9e–g ). These data identified PMLd327-344 as a mutant resistant to USP11-induced deubiquitination. 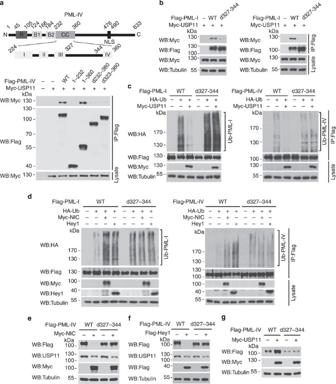Figure 9: Generation of a USP11-resistant mutant of PML. (a) Mapping of the USP11-interacting region on PML. The domain organization of PML is shown on the top. Interaction of USP11 with indicated PML deletion mutants in transfected 293T cells was analysed by coimmunoprecipitation assay. (b) PML 327–344 is required for interaction with USP11. 293T cells transfected with indicated constructs were analysed by coimmunoprecipitation. Of note, the amounts of PML deletion mutants used in transfection were adjusted to achieve similar expression levels of various PML proteins. (c,d) USP11, NIC and Hey1 cannot regulate the ubiquitination of PML d327-344 mutant. Immunoprecipitation and/or western blot analysis of PML-I or PML-IV ubiquitination in U87 cells transfected with indicated constructs. (e–g) Western blot analysis of PML expression levels in U87 cells transfected with indicated constructs. Figure 9: Generation of a USP11-resistant mutant of PML. ( a ) Mapping of the USP11-interacting region on PML. The domain organization of PML is shown on the top. Interaction of USP11 with indicated PML deletion mutants in transfected 293T cells was analysed by coimmunoprecipitation assay. ( b ) PML 327–344 is required for interaction with USP11. 293T cells transfected with indicated constructs were analysed by coimmunoprecipitation. Of note, the amounts of PML deletion mutants used in transfection were adjusted to achieve similar expression levels of various PML proteins. ( c , d ) USP11, NIC and Hey1 cannot regulate the ubiquitination of PML d327-344 mutant. Immunoprecipitation and/or western blot analysis of PML-I or PML-IV ubiquitination in U87 cells transfected with indicated constructs. ( e – g ) Western blot analysis of PML expression levels in U87 cells transfected with indicated constructs. Full size image Next, we tested the functional consequences of Hey1 overexpression or USP11 depletion in cells stably expressing wild-type PML or USP11-resistant PML. Remarkably, while Hey1 overexpression or USP11 depletion efficiently blocked the expression and anti-proliferation/migration/invasion effects of wild-type PML in U251 cells, they failed to alter the expression and functions of PMLd327-344 mutant ( Fig. 10a,b ). Similarly, NIC overexpression, Hey1 overexpression or USP11 knockdown drastically potentiated the self-renewal capability of GBM9 cells stably expressing wild-type PML, but they exerted only minor effects in cells expressing PMLd327-344 ( Fig. 10c,d ). These data indicate that PML is a major effector of the Notch/Hey1/USP11 axis in regulating the malignancy of GBM and GICs. 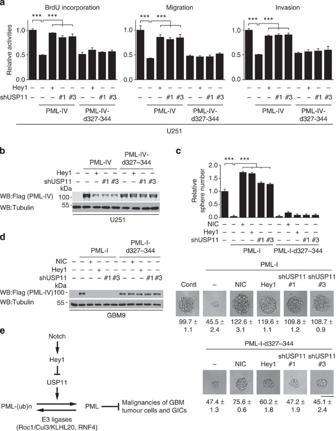Figure 10: The effects of Notch/Hey1 and USP11 on GBM and GIC are dependent on PML. (a) Proliferation, migration and invasion assays of U251 cells stably expressing indicated constructs. (b,d) Western blot analysis of PML expression in U251 and GBM9 cells stably expressing indicated constructs. These stable lines were used for experiments shown inaandc. Of note, to generate stable lines expressing comparable levels of wild type and mutant PML proteins, a higher titre of PML-IV-d327-344-expressing lentivirus was used for infection. (c) Sphere-forming assay of GBM9 cells stably expressing indicated constructs. Representative images of GIC neurospheres and their diameters (represented as mean±s.d. of 3 independent experiments, 30 neurospheres per group per experiment) are indicated on the bottom. Scale bars, 100 μm. Data in panelsaandcare mean±s.d. (***P<0.001 byt-test) of three independent experiments. (e) Schematic presentation of the Notch-induced PML degradation pathway and its functions in GBM. Figure 10: The effects of Notch/Hey1 and USP11 on GBM and GIC are dependent on PML. ( a ) Proliferation, migration and invasion assays of U251 cells stably expressing indicated constructs. ( b , d ) Western blot analysis of PML expression in U251 and GBM9 cells stably expressing indicated constructs. These stable lines were used for experiments shown in a and c . Of note, to generate stable lines expressing comparable levels of wild type and mutant PML proteins, a higher titre of PML-IV-d327-344-expressing lentivirus was used for infection. ( c ) Sphere-forming assay of GBM9 cells stably expressing indicated constructs. Representative images of GIC neurospheres and their diameters (represented as mean±s.d. of 3 independent experiments, 30 neurospheres per group per experiment) are indicated on the bottom. Scale bars, 100 μm. Data in panels a and c are mean±s.d. (*** P <0.001 by t -test) of three independent experiments. ( e ) Schematic presentation of the Notch-induced PML degradation pathway and its functions in GBM. Full size image Our study provides the first explanation of the molecular mechanism of PML deubiquitination. We demonstrated that USP11 deubiquitinates and stabilizes PML. The biological significance of this deubiquitination event is highlighted by the finding of USP11 downregulation in glioma, especially in grade IV GBM. Furthermore, this USP11 downregulation correlates with PML downregulation. At a functional level, the USP11/PML axis elicits inhibitory effects on multiple malignant characteristics of GBM, including proliferation, migration and invasion. Our study therefore uncovers the tumour suppressive effect of USP11-dependent PML stabilization. We further showed that USP11 is transcriptionally repressed by the Notch effector Hey1. Notch signalling is aberrantly activated in GBM and orchestrates the malignant traits of GBM and GICs, but current knowledge regarding the downstream players of Notch in GBM remains limited [43] . Our discovery of a link of USP11-dependent PML stabilization to the Notch/Hey1 axis highlights the significant contribution of this pathway to GBM malignancy. Indeed, using gain-of-function and loss-of-function approaches and the expression of a USP11-resistant PML mutant, we provide preclinical evidence showing that this PML degradation pathway is a part of the Notch programme to potentiate GBM proliferation, transformation and tumour growth in vivo , as well as GIC self-renewal, chemoresistance and tumour-forming capacities. Clinically, Hey1 overexpression, indicative of activated Notch signalling, correlates with USP11 and PML downregulation in GBM patients, suggesting the existence of this pathway and its aberrant activation in GBM. Thus, our study provides a molecular mechanism for PML downregulation in GBM and reveals a relevance of this PML regulatory pathway to GBM pathogenesis ( Fig. 10e ). The impact of the Notch/Hey1/USP11/PML pathway may extend beyond GBM and GICs. In mouse forebrain development, inactivation of Notch signalling compromises NPC maintenance, leading to precocious neuronal differentiation [43] , [44] . Loss of PML, however, suppresses the differentiation of radial glial cells, a type of NPC, to committed progenitor cells [19] . The opposite effects of PML and Notch on NPC fate decision are consistent with the negative regulation of PML by Notch identified in this study. Thus, it is tempting to propose that the Notch-induced PML degradation pathway similarly acts on NPCs to affect their maintenance and differentiation. Notably, USP11, one component of this pathway, is preferentially expressed in the forebrain ( Supplementary Fig. 3a ), implying its role in the development of this brain region. Although PML plays an inhibitory role in the maintenance of NPCs and GICs, a beneficial effect has been observed in HSCs [16] , [45] . Given the complexity of stem/progenitor biology and the pleiotropic functions of PML, it is conceivable that PML could elicit such context-dependent effects. In line with this notion, a recent study reveals an unexpected, pro-survival role of PML in certain cellular settings [45] , opposing the well-established pro-apoptotic function of PML. Given the highly heterogenous nature of GBM, future studies are needed to determine the functions of the Notch/Hey1/USP11/PML axis in different GBM subtypes. Notably, in addition to the cell intrinsic programme and environmental milieu, the functional complexity of PML can also be ascribed to the expression of different PML isoforms [4] , [6] . Although our study indicates that most PML isoforms are stabilized by USP11, they do not exert completely equivalent impacts on GBM pathogenesis. For instance, PML-IV displays stronger suppressive effects than PML-I on GBM cell proliferation, migration and invasion, but weaker effects on GIC self-renewal. It is possible that different PML isoforms interact with distinct partners, thus resulting in context-dependent biological functions. We have elucidated the mechanism by which Hey1 represses USP11 promoter activity ( Fig. 5i ). Hey1 is recruited to USP11 promoter via interacting with Sp1, which binds GC-rich sequences embedded in the CpG island of the USP11 promoter ( Supplementary Fig. 7a ). Sp1 binding is known to protect DNA from de novo methylation [46] , [47] . Consistently, the CpG island in the USP11 promoter was hypomethylated in GBM cell line U87 and most GBM patient samples were analysed ( Supplementary Fig. 7b,c ). Since CpG island methylation interferes with PRC2–chromatin interaction [48] , [49] , [50] , [51] , [52] , the hypomethylated USP11 promoter allows PRC2 recruitment by Hey1. The PRC2 component EZH2 catalyses H3K27 trimethylation, leading to chromatin compaction and transcriptional repression. Thus, Hey1 functions as a transcriptional corepressor in USP11 transcription regulation and a complex crosstalk among transcriptional factors, histone modifiers and DNA methylation is involved in Hey1-mediated repression of USP11 . In summary, our study identifies a PML degradation pathway, in which the Notch effector Hey1 represses PML-specific DUB USP11 to potentiate PML ubiquitination and degradation. This pathway is manifested in glioma, hyperactivated in GBM and contributes to the malignant characteristics of GBM and GICs. Blockage of this pathway might be a therapeutic strategy for treating the aggressive GBM. Cell culture and transfection HeLa, 293T, 293FT, H4, T98G, U87 and U251 cells were obtained from the American Type Culture Collection and PML -null MEF cells were obtained form Hsiu-Ming Shih. HeLa, 293T, 293FT, H4, T98G and PML -null MEF cells were cultured in DMEM containing 10% FCS. U87 and U251 cells were cultured in MEM containing 10% FCS. GBM9 and GBM004 cells were derived from pathologically diagnosed human GBM specimens under the approval by The Ohio State University Institutional Review Board and informed consent was obtained from these subjects. GICs were isolated using a method as described [53] . In brief, tumours were dissociated using TrypLE Express (Invitrogen) and cultured in Neurobasal medium (Invitrogen) with B27 (Invitrogen), human recombinant leukaemia inhibitory factor (10 ng ml −1 ; Chemicon International), basic fibroblast growth factor (50 ng ml −1 ; PeproTech), epidermal growth factor (50 ng ml −1 ; Millipore), penicillin G (100 units ml −1 ), streptomycin (100 units ml −1 ) and L -glutamine (2 mM; Invitrogen). The cells were validated for the expression of CD133, and the characteristics of self-renewal, ability to form tumours in low numbers and multilineage differentiation. GICs were grown as tumour spheres in Neurobasal medium supplemented with B27, 2 mM L -glutamine, 100 units ml −1 penicillin G, 100 units ml −1 streptomycin, 20 ng ml −1 epidermal growth factor and 20 ng ml −1 basic fibroblast growth factor. Transfection was performed with Lipofectamine 2000 Reagent (Invitrogen). Antibodies and reagents Antibodies used in this study and the validation information are listed in Supplementary Table 1 . DAPT was from Enzo. Cycloheximide, TMZ and As 2 O 3 were purchased from Sigma. MG132 was obtained from Calbiochem. Immunofluorescent staining and high-throughput image analysis Cells were fixed and permeabilized with ice-cold methanol for 20 min and blocked with PBS buffer supplemented with 10% goat serum and 1% BSA for 1 h. Cells were incubated with primary antibody ( Supplementary Table 1 ) at 4 °C for overnight and then with fluorescein isothiocyanate-conjugated secondary antibody together with 1 g ml −1 4′,6-diamidino-2-phenylindole (DAPI) for 1 h. For high-throughput quantifying the number and fluorescent intensity of PML-NBs, cells were examined by a Cellomics Arrayscan HT fluorescence microscope with a × 20 objective lens (Thermo Scientific). Images were acquired by a Cellomics Spot Detector Bioapplication program and analysed by a Cellomics vHCS:View software. DAPI signal was used for object selection. To correct plate-to-plate variation, the raw data were normalized with positive control (KLHL20 shRNA) and negative control (luciferase shRNA), which were included in each plate. Scores derived from two independent experiments in which each shRNA was performed in triplicate were averaged and plotted using the mean score of luciferase shRNA as 1. For quantifying PML-NBs in cells expressing various constructs, cells were examined by an epifluorescent microscope (1 × 71; Olympus) equipped with a camera (F-View II; Olympus) and controller software (analysis LS Research; Olympus). The number of PML-NBs per cell was quantified by ImageJ software using the function of Analyze Particles. Plasmid constructs Plasmids encoding myc-KLHL20, HA-ubiquitin, His-ubiquitin, myc-Cul3, myc-Roc1, HA-PML-I, HA-PML-IV, Flag-PML-I, Flag-PML-IV and Flag-PML-I-3KR were described previously [15] , [54] . The construct for NIC [55] was obtained from Ming-Zong Lai. Complementary DNAs for wild-type USP11 and C275/283S mutant were obtained from Winston CY Yu and then subcloned to pRK5myc, pCMV and pVL1393myc. The resistant USP11 construct was generated by site-directed mutagenesis. Hey1 cDNA was amplified by reverse transcriptase–PCR and subcloned to pRK5F and pBybe-myc. Various PML and USP11 deletion mutants were generated by PCR or ligation-mediated PCR. To clone USP11 promoter, a DNA fragment corresponding to nucleotides from −1,285 to +354 of the human USP11 gene was amplified from the genomic DNA of U87 cells and inserted to pGL3-based vector. Promoter mutant constructs were generated by site-directed mutagenesis. All constructs were verified by DNA sequencing. RNA interference and lentivirus transduction Lentivirus-based shRNA constructs were obtained from National RNAi Core Facility, Taiwan. The siRNAs to Sp1, Hey1 and Notch1 were obtained from Dharmacon. The target sequences of various shRNAs and siRNAs are listed in Supplementary Table 2 . Lentivirus generation and transduction were described previously [15] . Real-time reverse transcriptase–PCR analysis Quantitative real-time PCR analysis was performed using the Power SYBR Green PCR Master kit (Applied Biosystems). The sequences of various PCR primers are listed in Supplementary Table 2 . Amplification was performed on Roche LightCycler 480 system. Methylation-specific PCR and bisulphite sequencing Bisulphite modification of genomic DNA was performed using the EZ DNA Methylation Kit (Zymo Research). For MS–PCR, primers used for the methylated and unmethylated USP11 promoter are listed in Supplementary Table 2 . Genomic DNA from U87 cells treated in vitro by Sss1 methyltransferase (New England Biolabs) was used as a positive control, and normal human blood DNA was used as a negative control. For bisulphite sequencing, two pairs of primers used for amplifying USP11 promoter CpG island are listed in Supplementary Table 2 . The PCR products were cloned and individual clone was sequenced and evaluated using the BIQ Analyzer software. Protein analysis Cell extraction was performed with RIPA lysis buffer containing 50 mM Tris (pH 8.0), 0.15 M NaCl, 1% NP-40, 1% sodium deoxycholate, 0.1% SDS, 1 mM phenylmethyl sulphonyl fluoride, 1 μg ml −1 aprotinin and 1 μg ml −1 leupeptin. In experiments shown in Supplementary Fig. 2c,e , 5 μM N-ethylmaleimide (NEM) was added to the lysis buffer. Immunoprecipitation using cell lysates containing equal amounts of proteins was performed as described previously [56] . For in vitro pull-down analysis, Flag-PML-I was purified from baculovirus by anti-Flag agarose beads and eluted by Flag-peptide. Recombinant myc-USP11 was separately purified from baculovirus using c-myc AD agarose beads (Santa Cruz). The beads were incubated with purified Flag-PML-I for 1 h in binding buffer containing 20 mM Tris (pH 7.5), 150 mM NaCl, 1% NP-40, 0.1% SDS and 1% sodium deoxycholate and bound proteins were analysed by western blot. Full western blot images are shown in Supplementary Figs 8–13 . In vitro deubiquitination assay PML was first ubiquitinated in vitro essentially as described previously [15] . In brief, the purified Roc1–Cul3–KLHL20 complex bound on glutathione-sepharose beads was incubated with 200 ng of Flag-PML-I recombinant protein at 37 °C for 1.5 h in 20 μl reaction mixture containing 50 mM Tris (pH 7.5), 1 μM ubiquitin aldehyde, 20 μM MG132, 5 mM MgCl 2 , 2 mM ATP, 2 mM NaF, 1 mM dithiothreitol, 10 μg ubiquitin, 10 mM creatine phosphate, 500 ng creatine kinase, 40 ng yeast E1 enzyme and 500 ng E2 enzyme (UbcH5a). The reaction products were inactivated by heating for 15 min at 70 °C, and then incubated with baculovirally purified USP11 or its mutant in 40 μl deubiquitination reaction buffer containing 100 mM HEPES (pH 7.4), 500 mM NaCl, 100 mM MgCl 2 , 100 mM dithiothreitol and 10 mM ATP at 37 °C for 2 h. Reaction products were analysed by western blot. In vivo deubiquitination Cells transfected with various constructs together with HA-ubiquitin and Flag-PML were treated with 1 μM MG132 for 16 h and then lysed with RIPA lysis buffer supplemented with 1 μM MG132. Lysates were used for immunoprecipitation with anti-Flag antibody, followed by western blot with anti-HA antibody. Alternatively, cells expressing control or USP11 shRNA were transfected with His-ubiquitin and treated with 1 μM MG132. Cells were lysed by buffer A (6 M guanidine-HCl, 0.1 M Na 2 HPO 4 /NaH 2 PO 4 (pH 8.0) and 10 mM imidazole), and lysates were incubated with Ni-NTA agarose for 2 h at 4 °C. The beads were washed twice with buffer A/TI (1 vol buffer A: 3 vol buffer TI (25 mM Tris–HCl, pH 6.8 and 20 mM imidazole)), and five times with buffer TI, and then analysed by western blot. In all experiments, equal expression of HA-ubiquitin or His-ubiquitin was verified by western blot analysis. Apoptosis assay GBM9 derivatives (2 × 10 5 ) were pretreated with 25 μM DAPT or dimethylsulphoxide for 24 h and then with 25 μM TMZ for 48 h. Neurospheres were dissociated with Accutase (Millipore) and apoptotic cells were assayed by Annexin V kit (BD Pharmingen). Cell assays Cell proliferation was assayed using Cell Proliferation ELISA BrdU kit (Roche). In brief, 1 × 10 4 cells were seeded on plate and 5-bromo-2′-deoxyuridine was added to culture medium at 18 h after plating. 5-bromo-2′-deoxyuridine labelling was proceeded for 1 h before cell harvest. Transwell migration and invasion assays were performed essentially as described [56] . In brief, 2 × 10 4 cells were seeded on Transwell plate and incubated in culture medium for 6 h (for migration assay) or 18 h (for invasion assay). To distinguish migration/invasion effect from proliferation effect, the same number of cells was seeded on a regular culture plate. At the end of incubation, cells that had migrated onto the lower membrane surface of the Transwell plate were fixed with 4% formaldehyde, stained with DAPI and counted. The cell number was normalized with that appearing in the regular plate. For proliferation, migration and invasion assays, all data are presented as relative activities with the untreated control group as 1. Luciferase and ChIP assays For luciferase assay, cells were cotransfected with pGL3-based reporter construct and pCMV-renilla. Forty hours after transfection, luciferase activity in cell lysate was assayed by the Dual Luciferase Reporter Assay System (Promega). The relative promoter activity was expressed as the fold change in firefly luciferease activity after normalization to the renilla luciferase activity. ChIP assays were performed as described previously [15] . In brief, cells were fixed with 1% formaldehyde and processed for ChIP with various antibodies or normal mouse antiserum IgG (as a control). Enrichment of promoter binding levels was analysed by quantitative PCR, normalized by a negative control (located at a distal region of Hey1 promoter without E box- and Sp1-binding site), and expressed as fold increase over the control. The PCR primers for ChIP analysis are listed in Supplementary Table 2 . Tissue specimens and IHC analysis Freshly isolated human GBM specimens and benign tumour tissues (for MS–PCR) were obtained from Tri-service General Hospital, Taiwan. In addition, a human brain tumour microarray (for IHC) was obtained from Biomax Inc. Studies involving these tissues were approved by the Institutional Review Boards at Tri-Service General Hospital and Academia Sinica and informed consent was obtained from all subjects. For IHC analysis, antigen retrieval was performed by heat denaturation of paraffin sections with 10 mM sodium citrate buffer (pH 6.0) for 30 min. Endogenous peroxidase activity was blocked by incubation in 3% H 2 O 2 at room temperature for 20 min and nonspecific binding was blocked by Avidin/Biotin Blocking kit (Invitrogen). The slides were incubated with anti-Hey1 (1:100), anti-PML (1:100) or anti-USP11 (1:100) antibody in PBS containing 10% goat serum at room temperature for 2 h. The bound antibody was detected by biotinylated anti-mouse/rabbit IgG followed by peroxidase-labelled streptavidin and visualized with 3,3′-diaminobenzidine in chromogen solution (Dako LASB kit). The sections were counterstained with haematoxylin. The IHC staining was scored as negative/weak positive (score 0), moderate positive (score 1+) and strong positive (score 2+) based on percentage of cells staining positive and staining intensity. Samples with score 2+ are defined as high expression and those with score 1+ and score 0 are defined as low expression. Soft agar colony formation and neurosphere formation assays For assaying colony formation in soft agar, 2 × 10 4 U87 or U251 cell derivatives were resuspended in 0.3% top agar. Colony formed after 4 weeks were stained by crystal violet and the colony number was quantified by ImageJ software. For assaying neurosphere formation, GICs infected with lentivirus expressing various cDNAs and/or shRNAs were plated on 96-well plates at a density of 1 cell per well and cultured in GIC culture medium with or without DAPT. After 10 days, the percentage of wells containing neurospheres was quantified and neurospheres were imaged by a light microscope (1 × 71; Olympus) equipped with a camera (F-View II; Olympus). All data were normalized with the untreated control group. Intracranial tumour assays All mice experiments were conducted with approval from the Experimental Animal Committee, Academia Sinica, and followed guidelines of ethical regulations. For intracranial injection, 7- to 9-week-old, male BALB/c nude mice were anaesthetized and placed into stereotactic frame. The burr hole in the skull was drilled 1 mm anterior and 1.8 mm lateral to the bregma. Cells were resuspended in PBS and injected at a depth of 3.0 mm from the surface of the brain. For pathological analysis, three animals per group were used. At the appropriate days after injection, the mice were deeply anaesthetized and brains were fixed by intracardiac perfusion with 4% paraformaldehyde followed by a 12 h of immersion fixation. Brains were sectioned and paraffin-embedded sections were processed for haematoxylin and eosin staining. Bioinformatics Human USP11 tissue expression data were retrieved from the Genevestigator database ( https://www.genevestigator.com/gv/ ) using the Anatomy function. Microarray data derived from Human 133_2 (Human Genome 47k array) Array Platform were downloaded and output as a Heatmap-Tree with the Log2 display pattern. Transcriptional factor-binding site prediction was performed with the PROMO 3.0 program ( http://www.alggen.lsi.upc.es/cgi-bin/promo_v3/promo/promoinit.cgi?dirDB=TF_8.3 ). A region from 3,000 bp upstream to 3,000 bp downstream of the transcriptional start site of USP11 gene was queried and all human transcription factors and all sites were selected for analysis. Microarray and clinical data of glioma patients were obtained from the REMBRANDT database ( http://www.rembrandt.nci.nih.gov/ ). Gene expression values derived from the Affymetrix U133 plus 2.0 Array Platform for USP11 were downloaded for all glioma samples and normal samples through the Advanced Search function and via the caINTEGRATOR homepage. ChIP-seq data were retrieved from the UCSC Genome Browser ( http://www.genome.ucsc.edu/ ) assembled on March 2006. The locations of transcription factors bound to human USP11 5′-regulatory region were displayed by the Encode Transcription factor ChIP-seq function. Statistical analysis The two-tailed, Student’s t -test was used to compare between two groups and expressed as P -values. * P <0.05, ** P <0.01 and *** P <0.001. The Fisher’s exact test was used to compare the dichotomous variables. The Kaplan–Meier estimation and the log-rank test were used to compare the survival difference. All data were derived from independent experiments and the cells were not pooled across experiments. How to cite this article: Wu, H.-C. et al. USP11 regulates PML stability to control Notch-induced malignancy in brain tumours. Nat. Commun. 5:3214 doi: 10.1038/ncomms4214 (2014).